Implementing a strand of a scalable fault-tolerant quantum computing fabric With favourable error thresholds and requiring only nearest-neighbour interactions on a lattice, the surface code is an error-correcting code that has garnered considerable attention. At the heart of this code is the ability to perform a low-weight parity measurement of local code qubits. Here we demonstrate high-fidelity parity detection of two code qubits via measurement of a third syndrome qubit. With high-fidelity gates, we generate entanglement distributed across three superconducting qubits in a lattice where each code qubit is coupled to two bus resonators. Via high-fidelity measurement of the syndrome qubit, we deterministically entangle the code qubits in either an even or odd parity Bell state, conditioned on the syndrome qubit state. Finally, to fully characterize this parity readout, we develop a measurement tomography protocol. The lattice presented naturally extends to larger networks of qubits, outlining a path towards fault-tolerant quantum computing. Quantum error correction is an essential step towards realizing scalable quantum computers. Theoretically, it is possible to achieve arbitrarily long protection of quantum information from corruption due to decoherence or imperfect controls, so long as the error rate is below a threshold value [1] , [2] . However, most of the initial fault-tolerant quantum computing proposals were purely theoretical studies that would be impractical to implement in a physical system. Knill’s C4/C6 architecture [3] showed that it was possible to have a pseudo-threshold as high as 3% but with very long-range interactions. The two-dimensional surface code (SC) is a topological error-correcting code [4] , [5] that achieves high error thresholds ~\n1% in a two-dimensional lattice of qubits supporting nearest-neighbour interactions [6] , [7] . With ongoing improvements to coherence times [8] , [9] , [10] , [11] , and with gate [12] , [13] and readout fidelities [14] , [15] , [16] at or approaching relevant threshold values, superconducting qubits are prime candidates for scaling up towards a fault-tolerant architecture. Our scheme for building a network of superconducting qubits employs microwave resonators as the links, as it has been shown that resonators can be used as quantum buses to mediate interactions between qubits [17] , and that multiple resonators can be coupled to a single qubit [18] . In the future, larger superconducting qubit systems and networks will also leverage circuit integration techniques that come along with a solid-state architecture. The original SC layout comprises qubits arranged in a square lattice [5] with the qubits in the lattice coming in two distinct flavours, either code qubits, which carry logical information, or syndrome qubits, which are used to measure stabilizer operators of surrounding code qubits. Performing a round of error correction in the SC consists of applying controlled-NOT (CNOT) gates to map the parity of the surrounding code qubits into the states of the syndrome qubits, which are then measured to determine the plaquette parities. Using superconducting resonators as the links of the lattice, it is possible to construct a SC architecture using superconducting qubits at each vertex along with the ability to couple a single qubit to four resonators. As it is also important to be able to read out and address the qubits individually, this may require an additional fifth resonator per qubit. A layout proposed by DiVincenzo [19] allows for the number of resonators per qubit to be reduced to two (three with readout). However, each code and syndrome qubit in this scheme is replaced by four qubits, which results in a fourfold increase in the number of two-qubit gates. Here we introduce an optimal layout for implementing the SC on a two-dimensional lattice that does not carry additional overhead as in the original DiVincenzo proposal. In this work, we demonstrate a subsection of this optimized lattice using three transmon qubits, in which two independent outer code qubits are joined to a central syndrome qubit via two independent bus resonators. By combining all-microwave high-fidelity single- and two-qubit nearest-neighbour entangling gates, with high-fidelity measurement of the syndrome qubit, we deterministically measure the parity of the code qubits. This protocol is tested in the case of a superposition of the code qubits, and we are able to detect the outer code qubits in either an even or odd parity Bell state, conditioned on the syndrome state. As a full characterization of this parity detection, we implement a measurement tomography protocol to obtain a fidelity metric (90% for odd and 91% for even). Our results reveal a straightforward path for expanding superconducting circuits towards larger networks for the SC and eventually a primitive logical qubit implementation. Modified lattice for SC with superconducting qubits We introduce a direct one-to-one mapping of the SC to a two-dimensional lattice ( Fig. 1 ) that does not carry the additional overhead of qubits and gates as in the original proposal by DiVincenzo [19] . Rather than requiring 12 qubits to demonstrate a half-plaquette strand operation on the surface fabric, this arrangement allows such an achievement with just 3 qubits (details about the mapping are given in the Methods). Syndrome qubits can be used as either X -parity checks (red circles) or Z -parity checks (green circles) of four surrounding code qubits (blue circles). The five-qubit block consisting of X ( Z )-syndrome and four surrounding code qubits defines a unit cell X ( Z )-plaquette. 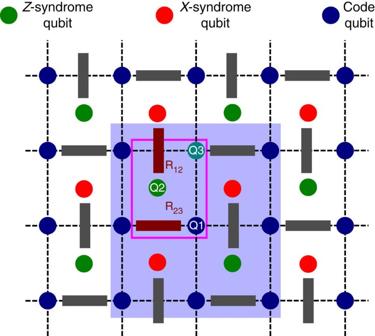Figure 1: Implemented two-dimensional SC layout. Lattice of nearest-neighbour qubits for realizing the SC. The lattice contains three flavours of qubits, code (blue circles),X-syndrome (red circles) andZ-syndrome (green circles) qubits. The lattice is composed of two types of plaquettes, anX-plaquette (square enclosing a redX-syndrome qubit) and aZ-plaquette (square enclosing a greenZ-syndrome qubit). Critical to the SC is performing CNOT operations between code qubits and their neighbouring syndrome qubits, followed by measuring theZ- andX-syndrome qubits to determine the parity of the code qubits. Bus resonators that link qubits are denoted by grey bars and each qubit need only connect to two bus resonators instead of the required four in the strict square lattice approach. The smallest logical qubit is shown in the shaded blue area, made up of four plaquettes. The half-plaquette device studied here is enclosed in the pink square and comprises three qubits (Q1, Q2, Q3) and two bus resonators R12and R23. Note that Q3 is also a code qubit, but coloured in teal for clarity to be distinguished from Q1. Figure 1: Implemented two-dimensional SC layout. Lattice of nearest-neighbour qubits for realizing the SC. The lattice contains three flavours of qubits, code (blue circles), X -syndrome (red circles) and Z -syndrome (green circles) qubits. The lattice is composed of two types of plaquettes, an X -plaquette (square enclosing a red X -syndrome qubit) and a Z -plaquette (square enclosing a green Z -syndrome qubit). Critical to the SC is performing CNOT operations between code qubits and their neighbouring syndrome qubits, followed by measuring the Z - and X -syndrome qubits to determine the parity of the code qubits. Bus resonators that link qubits are denoted by grey bars and each qubit need only connect to two bus resonators instead of the required four in the strict square lattice approach. The smallest logical qubit is shown in the shaded blue area, made up of four plaquettes. The half-plaquette device studied here is enclosed in the pink square and comprises three qubits (Q1, Q2, Q3) and two bus resonators R 12 and R 23 . Note that Q3 is also a code qubit, but coloured in teal for clarity to be distinguished from Q1. Full size image An advantage of our lattice architecture is that it is commensurate with experiments already demonstrated, where a single qubit can be coupled to two separate resonators [18] , a single bus has been used to couple up to three qubits [20] , and an independent readout can be used to measure a single qubit that has been entangled with a separate qubit via a bus resonator [21] . The experiments presented in this article are performed effectively on a ‘half-plaquette’ subsection, consisting of three qubits (all with individual readout resonators) and two bus resonators, depicted by the pink square of Fig. 1 , where we demonstrate all necessary gate operations and measurements that constitute the SC protocol. Physical subsection and control characterization The half-plaquette device ( Fig. 2a ) contains three single-junction transmon qubits connected by two coplanar waveguide (CPW) resonators serving as the buses, and each qubit is coupled to its own separate CPW resonator for independent readout and control. Here we label the code qubits Q1 and Q3, and the middle qubit Q2 serves as the syndrome. A simplified control and readout diagram is also shown in Fig. 2a , with all microwave sources for single- and two-qubit gates and independent readout indicated. The syndrome Q2 is read out with the assistance of a Josephson parametric amplifier (JPA) [16] , [22] for high-fidelity single-shot state discrimination, which is a critical component for demonstrating the SC parity check protocol. All device parameters, relevant coherence times and a complete schematic are given in the Methods. All single-qubit controls are performed in 40 ns and characterized to >99.7% average gate fidelity via simultaneous randomized benchmarking [23] (see Methods). 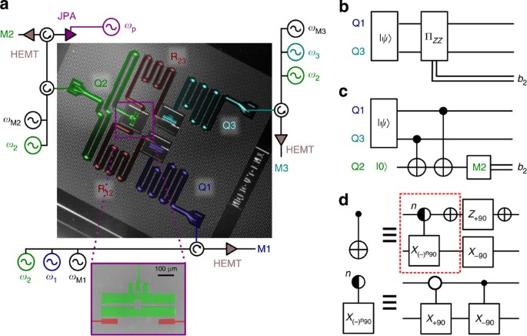Figure 2: Half-plaquette device schematic and parity check quantum circuits. (a) The optical image of the half-plaquette device shows in false colour all the different components of the device: three qubits, Q1 (blue), Q2 (green) and Q3 (teal), each with individual readout resonators, and two bus resonators (maroon) R12and R23. Each transmon qubit (zoom view inset) is independently addressed via its corresponding readout resonator, with single-qubit gates applied on resonance with each qubit atωi,iε[1, 2, 3] and readout performed at the measurement frequenciesωMi. Whereas Q1 and Q3 readout signals are only amplified through HEMTs, the Q2 readout is reflected off a JPA stage first before going on to a HEMT. Two-qubit gates are performed in the cross-resonance scheme, applyingω2on both control qubits, Q1 and Q3. (b) The PCP for qubit Q1 and Q3 where theZ-parity operator ΠZZis applied, giving a single classical bit of informationb2(double lines indicate classical channel). (c) The quantum circuit which implements theZ-parity check consists of a pair of CNOT gates from the code qubits (Q1 and Q3) to the syndrome (Q2) followed by a measurement M2, which gives the classical bitb2. (d) The CNOT can be decomposed into theZX90gate and single-qubit rotations. Using the cross-resonance microwave interaction, we have at our disposal the gate combination boxed in dashed red, composed of aZX90followed by a NOT (orX) gate on the control qubit. Thenin the depiction of theZX90gate can be either 0 or 1, indicating the state-dependent rotation. Figure 2: Half-plaquette device schematic and parity check quantum circuits. ( a ) The optical image of the half-plaquette device shows in false colour all the different components of the device: three qubits, Q1 (blue), Q2 (green) and Q3 (teal), each with individual readout resonators, and two bus resonators (maroon) R 12 and R 23 . Each transmon qubit (zoom view inset) is independently addressed via its corresponding readout resonator, with single-qubit gates applied on resonance with each qubit at ω i , i ε[1, 2, 3] and readout performed at the measurement frequencies ω M i . Whereas Q1 and Q3 readout signals are only amplified through HEMTs, the Q2 readout is reflected off a JPA stage first before going on to a HEMT. Two-qubit gates are performed in the cross-resonance scheme, applying ω 2 on both control qubits, Q1 and Q3. ( b ) The PCP for qubit Q1 and Q3 where the Z -parity operator Π ZZ is applied, giving a single classical bit of information b 2 (double lines indicate classical channel). ( c ) The quantum circuit which implements the Z -parity check consists of a pair of CNOT gates from the code qubits (Q1 and Q3) to the syndrome (Q2) followed by a measurement M2, which gives the classical bit b 2 . ( d ) The CNOT can be decomposed into the ZX 90 gate and single-qubit rotations. Using the cross-resonance microwave interaction, we have at our disposal the gate combination boxed in dashed red, composed of a ZX 90 followed by a NOT (or X ) gate on the control qubit. The n in the depiction of the ZX 90 gate can be either 0 or 1, indicating the state-dependent rotation. Full size image At the crux of the SC protocol is the detection of the parity of the code qubits. Figure 2b shows the parity check protocol (PCP) in a circuit depiction on an arbitrary state of Q1 and Q3, with the parity being indicated through the classical detection of an indication bit, b 2 . The PCP is realized in a system of three qubits via the quantum circuit shown in Fig. 2c , where the parity of the Q1 and Q3 state is mapped on to the syndrome Q2 via two CNOT gates, between Q1 and Q2, Q3 and Q2, and then subsequently the classical indication bit b 2 is obtained via a quantum measurement of Q2. High-fidelity CNOT entangling gates are critical for the PCP. To realize these CNOTs in our device, we implement entangling ZX 90 gates using the cross-resonance interaction [24] , [25] . By driving Q1 (Q3) at the Q2 transition frequency ω 2 , we use a simple decoupling sequence [12] to implement the two-qubit Clifford generator ZX 90 gate between Q2 and Q1 (Q3). The ZX 90 gate is equivalent to a CNOT up to single-qubit rotations, as illustrated in Fig. 2d , and thus can be used interchangeably in the PCP. Both pairs of ZX 90 entangling gates are characterized with two-qubit Clifford randomized benchmarking. With a total gate time of 350 ns, the ZX 90 gate between Q2 and Q1 (Q3) is experimentally shown to have a gate fidelity of 0.962±0.002 (0.957±0.001). The fidelities are consistent with the gate and coherence times in the system. Further details about the gate tune-up, calibration and timescales can be found in the Methods. To determine the collective state of all qubits in the system, we can perform independent readouts of each qubit through the individually coupled resonators. The syndrome qubit, Q2, is read out dispersively with the JPA, pumped −4 MHz from the readout frequency ( ω M2 =2π·6.584 GHz) and an optimized single-shot assignment fidelity (with no preparation corrections, and defined in Methods) of 91% is achieved, although fluctuations on the order of 2–3% are observed. The code qubits are read out using the high-powered Josephson nonlinearity of the readout cavities [26] . Further detail and parameters about the readouts are given in the Methods. Distributed entanglement and parity measurement To observe the action of the gate portion of the PCP, in which CNOT (in our case ZX 90 ) gates are performed between the syndrome and the code qubits, it is insightful to perform tomographic reconstruction of the complete three-qubit system. State tomography in our system is achieved by correlating individual single shots of all three individual readouts [27] , M i , i ε[1,3]. 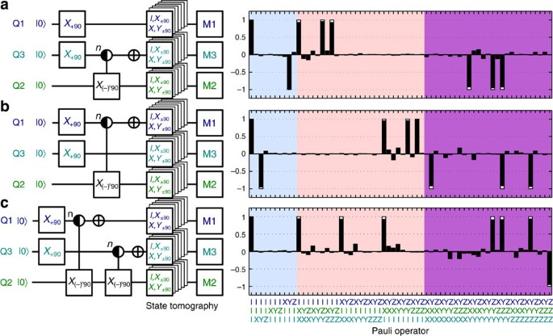Figure 3: Three-qubit state tomography via correlated single-shot readout. Building towards the action of the PCP on a superposition state of the code qubits (c), we also show the operation of entangling the syndrome Q2 with each of the data qubits Q1 (a) and Q3 (b). Reconstructed three-qubit state represented in Pauli state vector form (black filled bars, experiment, white bars in background, ideal) after entangling syndrome Q2 with,a, code qubit Q3 via aZX90two-qubit gate (entangled two-qubit state with fidelitystate~\n0.95), (b) code qubit Q1 via aZX90two-qubit gate (entangled two-qubit state with fidelitystate~\n0.95), (c) both code qubits Q1 and Q3 viaZX90between Q1 and Q2, and Q3 and Q2 simultaneously (which comprise performing the gate portion of the PCP) giving the maximally entangled three-qubit GHZ state (state~\n0.94). In the shown Pauli vector plots, the blue-, pink- and purple-shaded regions signify single-, two- and three-qubit Pauli operators, respectively. Figure 3 shows reconstructed three-qubit Pauli state vectors for the entanglement processes necessary for the PCP. In Fig. 3a , a ZX 90 entangling operation between the code qubit Q3 and the syndrome Q2 is implemented giving a state fidelity state =0.949±0.002 (SDP) 0.954±0.002 (raw), where SDP refers to a semi-definite program reconstruction of the state and raw reflects unconstrained inversion [28] . The difference between the SDP and raw estimates exceeds the statistical error estimated from the readout signal-to-noise and suggests that the main source of error in our experiment is systematic. We estimate that our systematic errors are of order ~\n2–3%. A rigorous error bound on fidelity in the presence of systematic noise is still the subject of future study [29] . In Fig. 3b , a ZX 90 entangling operation between Q1 and Q2 is implemented ( state =0.951±0.002 (SDP) 0.953±0.003 (raw)) and finally, in Fig. 3c both ZX 90 gates are applied simultaneously, generating a maximally entangled GHZ state of all three qubits ( state =0.935±0.002 (SDP) 0.942±0.003 (raw)). We thus show the ability to distribute entanglement across the full network, first between nearest-neighbour qubits Q3 and Q2 or Q1 and Q2, and then across the entire system with the GHZ state, spanning both bus resonators. Figure 3: Three-qubit state tomography via correlated single-shot readout. Building towards the action of the PCP on a superposition state of the code qubits ( c ), we also show the operation of entangling the syndrome Q2 with each of the data qubits Q1 ( a ) and Q3 ( b ). Reconstructed three-qubit state represented in Pauli state vector form (black filled bars, experiment, white bars in background, ideal) after entangling syndrome Q2 with, a , code qubit Q3 via a ZX 90 two-qubit gate (entangled two-qubit state with fidelity state ~\n0.95), ( b ) code qubit Q1 via a ZX 90 two-qubit gate (entangled two-qubit state with fidelity state ~\n0.95), ( c ) both code qubits Q1 and Q3 via ZX 90 between Q1 and Q2, and Q3 and Q2 simultaneously (which comprise performing the gate portion of the PCP) giving the maximally entangled three-qubit GHZ state ( state ~\n0.94). In the shown Pauli vector plots, the blue-, pink- and purple-shaded regions signify single-, two- and three-qubit Pauli operators, respectively. Full size image With the demonstrated high-fidelity ZX 90 gate primitives for the PCP, the next step is to observe the single-shot readout of the syndrome Q2 to signal the parity of the code qubits Q1 and Q3. We begin by obtaining a syndrome readout calibration histogram (a typical one is shown in Fig. 4a ). Then, we prepare the simple computational basis states, , , and , as inputs for the code qubits and observe the proper parity assignment via the PCP, shown via the M2 histograms in Fig. 4b . By thresholding the measurement outcomes of M2 based on the readout calibration traces, we reconstruct the state of Q1 and Q3 conditioned on M2 using standard quantum state tomography techniques (see Methods). In the case of the four computational states, we obtain fidelity of SDP =0.984, 0.987, 0.989, 0.909 and raw =0.975, 0.989, 0.999, 0.905, respectively. 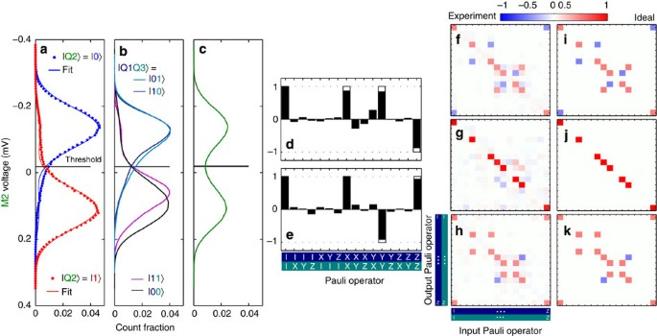Figure 4: Parity check experiment and non-nearest-neighbour pair entanglement generation. (a) Readout histograms of M2 having prepared Q2 in the stateandaveraged over all basis states for Q1 and Q3. (b) Readout histograms of M2 after applying the PCP when Q1 and Q3 are prepared in the four different basis states,(black),(teal),(blue),(purple). (c) Readout histogram of measurement M2 after applying the PCP when Q1 and Q3 are prepared in an equal superposition state. (d,e) Pauli state vectors of Q1 and Q3 conditioned on the single-shot measurement of Q2. In the case of Q2 in, state tomography confirms the odd (even) parity Bell state,with fidelity 0.89 (0.95). (f–k) Pauli transfer matrices of theZ-parity check measurement operation. Top (bottom) corresponds to the odd (even) projection and has a measurement fidelity of 0.90 (0.91). The central measurement operation corresponds to the unconditional map and has a fidelity of 0.968 with a map that is completely dephasing in the even and odd parity basis. Figure 4: Parity check experiment and non-nearest-neighbour pair entanglement generation. ( a ) Readout histograms of M2 having prepared Q2 in the state and averaged over all basis states for Q1 and Q3. ( b ) Readout histograms of M2 after applying the PCP when Q1 and Q3 are prepared in the four different basis states, (black), (teal), (blue), (purple). ( c ) Readout histogram of measurement M2 after applying the PCP when Q1 and Q3 are prepared in an equal superposition state. ( d , e ) Pauli state vectors of Q1 and Q3 conditioned on the single-shot measurement of Q2. In the case of Q2 in , state tomography confirms the odd (even) parity Bell state, with fidelity 0.89 (0.95). ( f – k ) Pauli transfer matrices of the Z -parity check measurement operation. Top (bottom) corresponds to the odd (even) projection and has a measurement fidelity of 0.90 (0.91). The central measurement operation corresponds to the unconditional map and has a fidelity of 0.968 with a map that is completely dephasing in the even and odd parity basis. Full size image A more complete stress test of the PCP is to observe its function on the maximal superposition state of the code qubits Q1 and Q3. The gate protocol now mimics that of the GHZ state generation from Fig. 3c , and over repeated state preparations and measurements of the syndrome, M2, we obtain a bi-modal histogram, indicating that instances of both parities exist ( Fig. 4c ). We observe the probabilistic entanglement of either the odd or even Bell states or conditioned on M2. For these conditioned entangled states, we find state fidelities of odd =0.891 (raw) 0.891 (SDP) and even =0.970 (raw) 0.948 (SDP). In an error-free situation, these fidelities should not exceed the assignment fidelity; however, due to systematic errors it is possible for these to deviate. The observed deviation between the assignment and state fidelity is within our estimate of systematic error. Nonetheless, the ability to generate these entangled states of non-nearest-neighbour qubits Q1 and Q3 in two separate bus resonators is a crucial element for scaling up towards larger quantum networks. Finally, to characterize the complete ideal projective nature of the PCP, we perform measurement tomography. This is accomplished via quantum process tomography of the code qubits, for which further details are given in the Methods. Conditioned on the measurement of the syndrome M2, we obtain the two maps for the odd and even parity projection operators shown in Fig. 4f,h (ideal maps are shown in Fig. 4i,k ). To quantify the performance of the PCP, we introduce a measurement fidelity metric that takes into account the full quantum dynamics of the measurement, including projection and back-action (see Methods for more details). We obtain a measurement fidelity of and . The loss in measurement fidelity corresponds mostly to the 91% assignment fidelity of M2, best illustrated by the unconditional map (shown in Fig. 4g ) having a measurement fidelity meas =0.968. It is important to note that all the gates used are calibrated and run to achieve these results without any Hamiltonian corrections for either single-qubit or two-qubit errors. An X -parity check is a simple extension through the appropriate application of single-qubit Hadamard pulses on the code qubits. The experiment described implements a subsection of the SC fault-tolerant architecture. By combining high-coherence transmon qubits, high-fidelity nearest-neighbour two-qubit gates and high-fidelity quantum non-demolition single-shot readout, we use a syndrome qubit to determine the parity of its neighbouring qubits. With this device, we demonstrate the versatility of superconducting qubits in the extended quantum bus architecture for application towards a larger fault-tolerant quantum computing device. Looking ahead, direct extensions to simple error detection and error correction demonstrations will be feasible with existing integration techniques and coherence levels. Overcoming integrated circuit engineering hurdles while preserving long coherence times should pave the way for larger surfaces for quantum error correction. During the completion of this manuscript, we became aware of similar work by Saira et al . [33] Mapping to SC The SC requires CNOT gates to be performed between the code and syndrome qubits. To optimize the fidelity of these gates, it is important to use a connective element (connector) to mediate a strong interaction between these qubits. For superconducting transmon qubits, the connections are typically achieved by capacitively coupling two (or more) qubits to a resonator. Since the SC is a two-dimensional geometry, connectors should not cross. The most straightforward layout of the SC is to have the qubits arranged on a square lattice, each connected to its nearest neighbours (see Fig. 5a ). This arrangement has considerable overhead, in that each qubit is attached to four connectors. For a realization in a transmon-based architecture it will require each qubit having at least four capacitive couplers (not including readout and control lines). As a result, a significant amount of the qubit charging energy will come from the presence of the couplers. 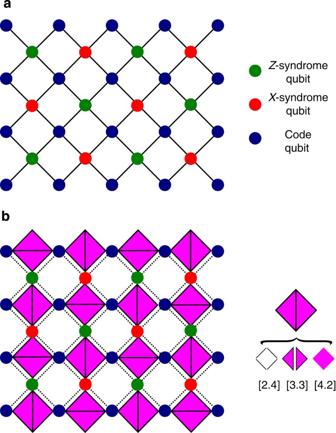Figure 5: Square lattice with connectors. (a) The conventional square lattice. Each qubit is connected to its four nearest neighbours. The lattice contains three flavours of qubits, code (blue circles),X-syndrome (red circles) andZ-syndrome (green circles) qubits. (b) Three kinds of connectivity: the pink squares shows a connector that is used to allow the application of gates required for the SC. This square can be made from four connectors, two connectors or a single connector. Figure 5: Square lattice with connectors. ( a ) The conventional square lattice. Each qubit is connected to its four nearest neighbours. The lattice contains three flavours of qubits, code (blue circles), X -syndrome (red circles) and Z -syndrome (green circles) qubits. ( b ) Three kinds of connectivity: the pink squares shows a connector that is used to allow the application of gates required for the SC. This square can be made from four connectors, two connectors or a single connector. Full size image Previously, DiVincenzo [19] has shown that it is possible to have a lattice that realizes the SC with each qubit attached only to two connectors. The DiVincenzo lattice is shown in Fig. 6 . In this lattice, each small square contains four qubits and is used to represent a single code or syndrome qubit. It is apparent that this arrangement has connectivity between the small squares that is equivalent to the standard square lattice. However, the mapping is inefficient in that it requires four qubits to represent a single qubit in the original SC and furthermore it requires as many as four CNOT operations spanning four connections (resonators) for the furthest reaches of adjacent squares to communicate. 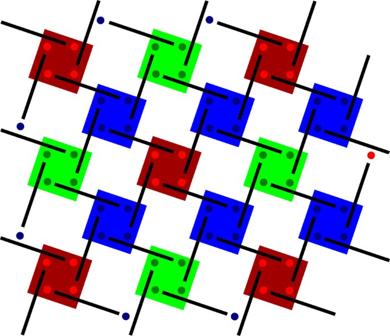Figure 6: Original skew-square lattice of DiVincenzo. Each code and syndrome qubit is represented by the small coloured squares, each containing four physical qubits. The black lines represent resonators (couplers). Figure 6: Original skew-square lattice of DiVincenzo. Each code and syndrome qubit is represented by the small coloured squares, each containing four physical qubits. The black lines represent resonators (couplers). Full size image Figure 5b shows three additional arrangements of connections in the square lattice. Connectors are located in every other square of the checkerboard, shown as pink, and each pink square represents either four, two or one connector. In the first case, the pink square is broken up into four connectors, each attached to two qubits and each qubit to four connectors, recovering Fig. 5a . We call this the [2,4] arrangement. The second arrangement is to divide the pink regions into two, with each connector joined to three qubits and each qubit attached to three couplers ([3,3] arrangement). Finally, the connector can be the entire pink square connecting four qubits with each qubit connecting only to two connectors ([4,2] arrangement). This final arrangement can easily been seen to achieve the desired simultaneous goals of having each qubit attached to just two connections while retaining the connectivity of the square lattice. As shown in Fig. 1 , the connector can be realized by using a resonator that connects to four qubits. The alternating horizontal and vertical lines inside the pink squares correspond precisely to the bus resonators. Two final points are worth discussing. First, note that the [4,2] arrangement is actually more connected than the square lattice, that is, diagonal neighbouring qubits can be coupled. This extra connectivity may be of some advantage, although it comes at the cost of reducing the isolation between these qubits. This is an unavoidable consequence of having more than two qubits per connector. Lastly, DiVincenzo’s lattice is a simple distortion, a skewing, of the [4,2] lattice. Our key observation can be thought of as seeing that his lattice can be directly mapped to the square lattice without having four qubits being used to represent just one qubit from the SC. Device fabrication The device is fabricated on a 720-μm thick silicon substrate. All superconducting CPW resonators are defined via optical lithography and subtractive reactive ion etching of a sputtered niobium film (200 nm thick). The three single-junction transmon qubits are patterned using electron-beam lithography, followed by double-angle deposition of aluminium, with layer thicknesses of 35 and 85 nm. Lift-off process is used to form the final junction structure. Device parameters The three transmon qubits ( i ε[1,3]) have transition frequencies {ω i }/2π={5.0388, 5.0080, 5.2286} GHz, with readout resonators at {ω R i }/2π={6.698, 6.585, 6.695} GHz, relaxation times { T 1( i ) }={24, 29, 20} μs, μs. The bus resonators are unmeasured but R 12 (R 23 ) is designed to resonate at 8 (8.5) GHz. The dispersive cavity shifts of the readout resonators are measured to be { χ i }/π={−2.0, −2.0, −2.3} MHz and the readout resonators have line widths { κ R i }/2π={443, 976, 793} kHz. All qubits have measured anharmonicities of ~\n−340 MHz. From the above, we calculate coupling strengths {| g i |}/2π={70, 67, 67} MHz to the readout resonators, which is consistent with electromagnetic simulations. Experimental set-up The half-plaquette device is cooled to 15 mK in an Oxford Triton dilution refrigerator. A full schematic of the wiring and experimental control hardware is depicted in Fig. 7 . Each qubit has its own dedicated readout line with an associated set of isolators and Caltech HEMT (noise temp ~\n6 K) amplifiers. Q2 is unique in that its readout signal is reflected off of a UC Berkeley JPA before going on to the isolator and high-electron mobility transistor (HEMT) chain. The device is housed in a light-tight Ammuneal cryoperm-shield that is coated throughout with a layer of lossy eccosorb (Emerson & Cuming CR-124). Besides explicit cryogenic attenuators at the different stages of the cryostat, all qubits are also attenuated at the lowest temperature stage with in-house eccosorb coaxial filters. 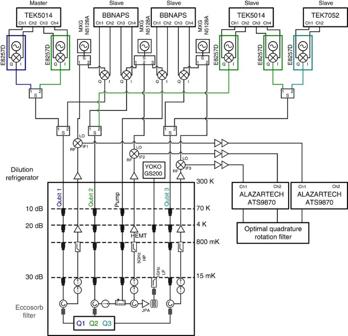Figure 7: Detailed schematic of experimental setup. Wiring scheme for all room temperature controls as well as internal configuration of Oxford Instruments Triton dilution refrigerator. Figure 7: Detailed schematic of experimental setup. Wiring scheme for all room temperature controls as well as internal configuration of Oxford Instruments Triton dilution refrigerator. Full size image Outside the cryostat, all microwave qubit control signals are generated via vector modulation combining off-the-shelf electronics. The microwave readout signals are pulse modulated using Arbitrary Pulse Sequencers built by Raytheon BBN Technologies. The readout signals are processed via two Alazartech ATS9870 acquisition cards. All single-shot readout traces are processed with various filters, down-sampling and an optimal quadrature rotation filter. The details of this full process, which is currently performed explicitly in the acquisition computer, is described in detail in parallel work [27] . As the devices scale up in the near term towards plaquette and logical qubit demonstrations, the multiple readout signals will need to be processed directly on Field-Programmable Gate Arrays and then correlated in post processing. Calibration sequences Complete tune-up of all microwave gates is accomplished using sets of automated repeated sequences. For single-qubit gates, the repeated calibration sequences are described in a previous publication [28] . The cross-resonance pulse amplitude is calibrated in close analogy to single-qubit amplitude calibrations. An odd number 2 N −1 of ZX 90 pulses are applied and the amplitude is adjusted so that for each N the expected signal is halfway between 0 and 1. Any amplitude miscalibrations lead to departures from this expected signal and are amplified for increasing N . In addition to amplitude, we must also calibrate the phase of the ZX 90 pulse between Q3 and Q2 (as well as Q1 and Q2). In our experiment, we use a separate microwave generator to supply the cross-resonance pulse on Q3 at the frequency of Q2. The phase of this microwave signal must be calibrated to match that of the microwave generator supplying the single-qubit pulses on Q2. This is done by applying the pulse sequence IY 90 ( ZU 180 IX ) N IX 90 . The U denotes the rotation axis defined by the second generator and the goal is to calibrate for an X -rotation. In the case of an X -rotation, we expect the signal to be halfway between 0 and 1 for each N and miscalibration of the phase leads to deviations that are amplified with increasing N . These methods provide a routine for automated calibration with high precision. In the experiments, all cross-resonance pulses were calibrated on a regular basis because of phase drift between the two microwave generators. Randomized benchmarking All single-qubit gates are 40-ns Gaussian-shaped microwave pulses (Gaussian width σ =10 ns) resonant with the transition frequencies of the qubits, with scaled derivative-of-Gaussian shapes applied on the quadrature channel to minimize leakage effects [30] . The gates are all autonomously calibrated with a set of repeated pulse experiments, correcting for: amplitude of X 90 and X gates, amplitude imbalance between X - and Y -rotations, mixer skew and derivative-of-Gaussian-shape parameter. Single-qubit gates are all independently characterized via Clifford [31] randomized benchmarking (RB) and summarized in Table 1 . To characterize the addressability error of the system, we perform simultaneous [23] RB, applying different sets of randomized single-qubit Clifford gates to all three qubits at the same time. These results are also summarized in Table 1 and essentially indicate that addressability errors are at the 0.1% error level. Table 1 Summary of single-qubit randomized benchmarking. Full size table The two-qubit ZX 90 gates for both pairs of qubits are composed as a two-qubit refocusing sequence previously described [32] and include shaped Gaussian turn-on (3 σ , σ =24 ns), a flat section and then a Gaussian turn-off, for a total gate time of 350 ns. The ZX 90 gates are tuned-up also using repeated pulse experiments (described in previous section). It is also important to note that the pair of two-qubit gates can be applied simultaneously, as they commute with one another. To characterize the gates, we generate two-qubit Clifford operations [12] and perform RB. The results for the two cases are shown in Fig. 8 , where we show the average fidelity decay over 35 different randomized two-qubit Clifford sequences. Analysing the decay curves gives us error per two-qubit Clifford gate of 0.058±0.003 for Q1 and Q2, and 0.065±0.002 for Q3 and Q2. We find that the reduced chi-square for these fits are 0.583 and 0.385, respectively. This demonstrates that the model is a faithful representation of the data. As each two-qubit Clifford gate is composed of 1.5 ZX 90 generators, we estimate the two-qubit ZX 90 gate errors to be 3.8 and 4.3%. 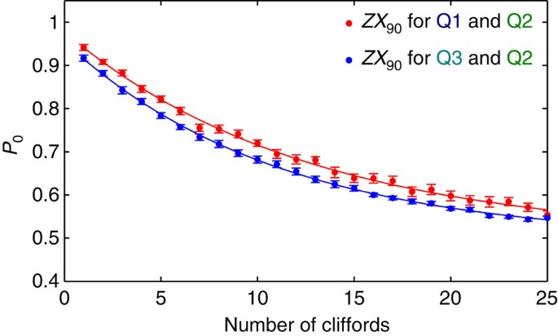Figure 8: Two-qubit randomized benchmarking. AverageP0, population of Q2 ground state, versus number of two-qubit Cliffords generated viaZX90gates between Q1 (Q3) and Q2 is shown as red (blue) circles. Experiments are performed randomizing over 35 different sequences of Cliffords. Fits to the RB experiment for Q1 (Q3) and Q2 are shown as solid red (blue) lines, from which we extract an error per two-qubit Clifford of 0.058±0.003 (0.065±0.002). Figure 8: Two-qubit randomized benchmarking. Average P 0 , population of Q2 ground state, versus number of two-qubit Cliffords generated via ZX 90 gates between Q1 (Q3) and Q2 is shown as red (blue) circles. Experiments are performed randomizing over 35 different sequences of Cliffords. Fits to the RB experiment for Q1 (Q3) and Q2 are shown as solid red (blue) lines, from which we extract an error per two-qubit Clifford of 0.058±0.003 (0.065±0.002). Full size image Readout characterization For this experiment, each qubit has its own measurement resonator. On Q1 and Q3 high-power readout was used and for Q2 a dispersive linear readout with a JPA was used. The readout was performed by using an integrating kernel that takes into account the response of the cavity (see ref. 27 for more details). This is important when most of the information is in the initial transients of the signal. The integration time for the experiment was 4 μs for the high-power readout and 2 μs for the dispersive readout with the JPA. Shown in Fig. 9 are typical histograms for the three readout channels averaged over all computational basis for the qubits not measured. 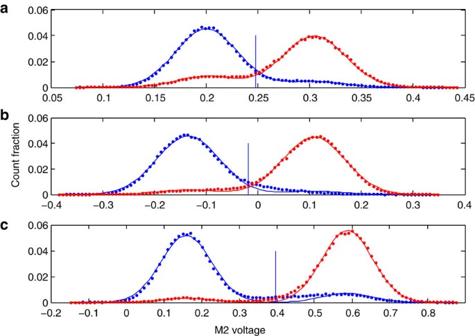Figure 9: Histogram of three independent readouts. (a) Histograms of the high-power readout used for Q1. (b) Histograms of the dispersive linear readout with a JPA for Q2. (c) Histograms of the high-power readout used for Q3. In all cases blue is preparing ground and red is excited. Solid lines are double-Gaussian fits to the histograms. Here we see that the assignment fidelity, defined by Figure 9: Histogram of three independent readouts. ( a ) Histograms of the high-power readout used for Q1. ( b ) Histograms of the dispersive linear readout with a JPA for Q2. ( c ) Histograms of the high-power readout used for Q3. In all cases blue is preparing ground and red is excited. Solid lines are double-Gaussian fits to the histograms. Full size image for the three channels is 0.84, 0.91 and 0.89, respectively. These are typical values and we see about a 2–3% fluctuation over the course of a typical experiment. By fitting a double-Gaussian model to the data, we find that the ratio of the undesired state to the desired state for Q1 prepared in the ground (excited) is 9.9% (22%), for Q2 5.7% (8.3%) and for Q3 13.7% (6.0%). We believe most of the error is due to the high-power nonlinear readout of Q1 and Q3 and is not due to the qubits being initialized in the wrong state. With no power applied to the Q1 and Q3 resonator, the assignment fidelity is 0.95 and the ratios of the two Gaussians are 5.6% when Q2 is prepared in the excited state and negligible when Q2 is prepared in the ground state. State tomography For state tomography we used the correlation method as described in ref. 27 . The single shots for each measurement resonator are correlated and from a set of complete post rotations we can use either linear inversion or an SDP (with constraints ρ ≤ and tr( ρ )=1) to reconstruct the state. The complete set of rotations used are { I , X , X +90 , X −90 , Y +90 , Y −90 } ⊗ n . Typically, 20,000 shots for each post rotation are used and we find that the statistical error in the measured voltages has signal-to-noise ratio (SNR) ~\n1 × 10 4 , 2 × 10 4 , 2 × 10 4 for the three measurement channels M1, M2, M3, respectively. The second-order correlators range in SNR from ~\n2 to 5 × 10 3 and the third order has SNR ~\n1,000. Using these and a bootstrapping method [28] we can estimate the state fidelity and the statistical error. The state fidelity is given by where ρ ideal is the ideal state and ρ noisy is the reconstructed state. We find that in all cases the fluctuations in the state fidelity from statistics is much smaller than the difference between the linear reconstruction and the SDP. Furthermore, we find typically the sum of all the negative eigenvalues in the three-qubit space to be <0.03. Measurement tomography An ideal Z -parity check can be described by the quantum operation where and the extra system is used to label the outcome of measurement of the syndrome qubit. In the noisy case this is represented by the operation and the goal of measurement tomography is to determine the conditional maps even ( ρ ) and odd ( ρ ). These quantum operations are completely positive but not trace preserving. By binning the results of the measurement on the syndrome qubit, tomography on the two-qubit subspace is performed by preparing a complete set of different input states and measurement bases via pre and post rotations, and reconstructing the operations from the measurement results. The complete set of rotations that we use are the same as those used in state tomography. We use both a linear reconstruction and a minimization to make the maps physical. For more details on how quantum process tomography can be performed, see ref. 28 . We use the Pauli transfer matrix [28] defined by to represent the measurement operations where P j s are the standard Pauli operators { I , X , Y , Z } ⊗ 2 . To quantify the measurement, we define the measurement fidelity by a generalization of the average fidelity. Since the measurement maps are not trace preserving, we need to use normalized outputs , and , where , tr refers to the trace norm and x ={even, odd}. Doing this gives Since the nullspace of a projection operation has measure zero and the noisy realization typically will also have a nullspace of zero measure, this integral is well defined. To compute this, we draw 150,000 different random states from the Fubini–Study measure and compute the average. One could also define a process fidelity by computing the state fidelity between normalized Choi matrices of the ideal and noisy operations however, for non-unitary processes there is no simple relationship between them. The unconditional map can be defined by tracing equation (5) over the syndrome qubit giving Since this is a quantum operation, the standard fidelity between quantum operations can be used. How to cite this article: Chow, J. M. et al . Implementing a strand of a scalable fault-tolerant quantum computing fabric. Nat. Commun. 5:4015 doi: 10.1038/ncomms5015 (2014).